PPARα-UGT axis activation represses intestinal FXR-FGF15 feedback signalling and exacerbates experimental colitis Bile acids play a pivotal role in the pathological development of inflammatory bowel disease (IBD). However, the mechanism of bile acid dysregulation in IBD remains unanswered. Here we show that intestinal peroxisome proliferator-activated receptor α (PPARα)-UDP-glucuronosyltransferases (UGTs) signalling is an important determinant of bile acid homeostasis. Dextran sulphate sodium (DSS)-induced colitis leads to accumulation of bile acids in inflamed colon tissues via activation of the intestinal peroxisome PPARα-UGTs pathway. UGTs accelerate the metabolic elimination of bile acids, and thereby decrease their intracellular levels in the small intestine. Reduced intracellular bile acids results in repressed farnesoid X receptor (FXR)-FGF15 signalling, leading to upregulation of hepatic CYP7A1, thus promoting the de novo bile acid synthesis. Both knockout of PPARα and treatment with recombinant FGF19 markedly attenuate DSS-induced colitis. Thus, we propose that intestinal PPARα-UGTs and downstream FXR-FGF15 signalling play vital roles in control of bile acid homeostasis and the pathological development of colitis. Bile acids are involved in nascent bile formation, cholesterol elimination and intestinal absorption of lipids and lipid-soluble molecules. Moreover, bile acids are increasingly recognized as signalling molecules in regulating energy homeostasis, inflammation and liver regeneration [1] , [2] , [3] , [4] , [5] , [6] . However, bile acids, some of which are toxic and can induce apoptotic and necrotic cell death, play important roles in promoting the development of diseases such as the well-defined cholestatic liver diseases. Thus, the concentration of bile acids must be strictly regulated to ensure a homeostasis state. Exposure of cells of the gastrointestinal (GI) tract to repeated high levels of bile acids is a vital risk factor for inflammatory bowel disease (IBD) and GI cancer [7] , [8] , [9] . Studies from both experimental animal models and clinical patients indicated that the levels of bile acids are increased in the conditions of IBD and colon cancer. The accumulation of taurocholic acid in the GI tract can aggravate colitis via regulating the compositions of intestinal flora, providing a potential mechanism that explains the high prevalence of IBD and colon cancer in the populations with western lifestyle and diet [10] . Moreover, repeated exposure of the colorectal epithelium to high physiological concentrations of bile acids is a major aetiologic factor in colorectal carcinogenesis [11] . Together, these lines of evidences strongly indicate that the long exposure of the GI tract to high levels of bile acids represents an important risk factor in the development of IBD and colon cancer. Thus, it is reasonable to propose that restoration of bile acid homeostasis may represent a useful approach to the therapy of IBD and even the prevention of colon cancer. However, the molecular mechanisms and pathways by which the bile acids are abnormally accumulated in IBD remain largely elusive. Farnesoid X receptor (FXR) is a master regulator maintaining the homeostasis of bile acids. In response to elevated levels of intracellular bile acids, FXR is activated to induce protective gene expression circuits against bile acid toxicity in the liver and intestine [12] . FXR induces small heterodimer partner (SHP) in the liver and FGF19 (FGF15 in rodents) that binds with liver fibroblast growth factor (FGF) receptor 4 (FGFR4) via an endocrine mode after its secretion from the intestine; both signal to inhibit CYP7A1, the rate controlling enzyme in the de novo synthesis of bile acids [13] , [14] , [15] , [16] . However, how the fine-tuned machinery is dysregulated and whether it is involved in pathological development of IBD remains to be answered. FXR, as a bile acid-activated transcriptional factor, senses the intracellular level of bile acids and shuts down genes involved in bile acid synthesis, influx and efflux. Thus, the intracellular concentration of bile acids is an important determinant of FXR transcriptional activity. Based on this consideration, we reasoned that it is crucial to clarify the intracellular disposition of bile acids for the better understanding of the role of dysregulated FXR signalling in IBD. In this study, we show that the activation of peroxisome proliferator-activated receptor α (PPARα)-UDP-glucuronosyltransferases (UGTs) axis reduces the intracellular levels of bile acids in the intestine, which compromises intestinal FXR-FGF15 signalling. This dysregulated signalling machinery leads to the continuous activation of liver CYP7A1 and thus the increased de novo synthesis of bile acids, and finally the accumulation of bile acids in the inflamed colon tissues. We further reveal that the intestinal PPARα-UGTs axis upstream of FXR-FGF15 pathway is an important determinant in the pathological development of dextran sulphate sodium (DSS)-induced colitis. Colitis induces bile acids accumulation in the colon Chronic DSS-induced murine colitis model was characterized by mucosal oedema, crypt distortion, a high level of leukocyte and polymorphonuclear infiltration, and dramatically increased expression of proinflammatory cytokines ( Supplementary Fig. 1 ). To assess how the overall bile acid profile was affected, bile acid composition analysis was carried out in different compartments of mice. A panel of bile acids in the liver, small intestine, colon, serum, urine and faeces of normal and DSS mice were detected ( Fig. 1 ). After analysing the individual bile acids in multiple compartments, a previously uncharacterized dysregulation feature of bile acids was identified in colitis. Compared with normal mice, the bile acid pool size was significantly increased in mice of DSS-induced colitis ( Fig. 1a ), which suggests an enhanced de novo synthesis of bile acids. A compartment-specific dysregulation pattern of bile acids was found. In general, the total levels of bile acids were lower in the serum in mice with colitis ( Fig. 1b ), while higher levels were observed in the gall bladder, small intestine, colon and faeces ( Fig. 1c–e ). In the small intestine, multiple unconjugated bile acids, including chenodeoxycholic acid (CDCA), deoxycholic acid (DCA), cholic acid (CA), ursodeoxycholic acid (UDCA), HDCA and β-muricholic acid (β-MCA), were decreased while the conjugated bile acids increased in colitis mice ( Fig. 1f ). Of particular interest, the inflamed colon showed a much higher concentration for most of bile acid species (including conjugates and free bile acids), supporting a specific intracellular accumulation of toxic bile acids species in the inflamed colon tissues. 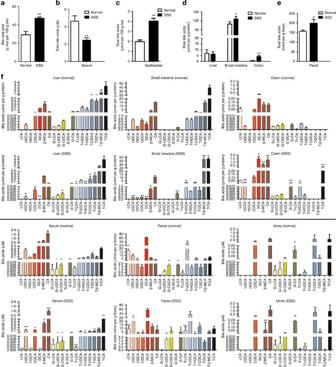Figure 1: DSS-induced colitis disrupts bile acids homeostasis. (a) Bile acid pool analysis. The bile acid pool size was analysed by measuring total bile acids in the whole enterohepatic system, including the liver, gall bladder and the entire small intestine and its contents, and the values were normalized by body weight. (b–e) Total amount of bile acids in individual compartments. (f) Compartmental individual bile acid profiles analysed by a UFLC-Triple-time of flight/MS analysis in the control and colitis mice. Results are mean±s.e.m of six mice, *P<0.05, **P<0.01 versus normal control, Student’st-test. CA, cholic acid; LCA, lithocholic acid; UDCA, ursodeoxycholic acid; CDCA, chenodeoxycholic acid; DCA, deoxycholic acid; MCA, muricholic acid; T, tauro-conjugated species; G, glycine-conjugated species. Figure 1: DSS-induced colitis disrupts bile acids homeostasis. ( a ) Bile acid pool analysis. The bile acid pool size was analysed by measuring total bile acids in the whole enterohepatic system, including the liver, gall bladder and the entire small intestine and its contents, and the values were normalized by body weight. ( b – e ) Total amount of bile acids in individual compartments. ( f ) Compartmental individual bile acid profiles analysed by a UFLC-Triple-time of flight/MS analysis in the control and colitis mice. Results are mean±s.e.m of six mice, * P <0.05, ** P <0.01 versus normal control, Student’s t -test. CA, cholic acid; LCA, lithocholic acid; UDCA, ursodeoxycholic acid; CDCA, chenodeoxycholic acid; DCA, deoxycholic acid; MCA, muricholic acid; T, tauro-conjugated species; G, glycine-conjugated species. Full size image Hepatic CYP7A1 is upregulated in DSS-induced colitis The result of increased bile acid pool size suggests an increased de novo synthesis of bile acids. The regulation pattern of hepatic CYP7A1, the rate-controlling enzyme in the de novo synthesis of bile acids, was thus examined. As expected, the hepatic expression of Cyp7a1 mRNA and protein content was significantly increased in colitis compared with that in control mice ( Fig. 2a,b ). In contrast, the hepatic expression of Cyp8b1 , Cyp7b1 and Cyp27a1 mRNAs was not significantly affected ( Fig. 2a ), consistent with the similar CA levels observed in the liver of the two groups. Little liver damage and inflammation was found in DSS-induced colitis mice ( Supplementary Fig. 2a–d ). Hepatic Hnf4α and Lrh-1 were proposed to function as important transcription factors in controlling bile acid synthesis and in the induction of Cyp7a1 by transactivating Cyp7a1 promoter activity [17] . Unexpectedly, both Hnf4α and Lrh-1 mRNA expression were markedly decreased in the liver of colitis mice ( Supplementary Fig. 2e ). These results indicate that the upregulation of hepatic Cyp7a1 is unlikely attributed to the activation of positive regulating signals in the liver. 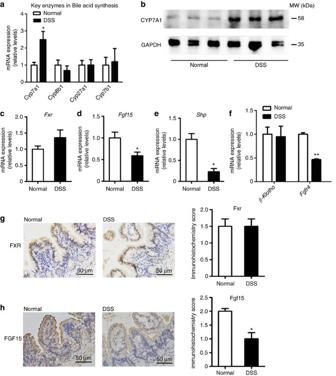Figure 2: The intestinal FXR-FGF15 signalling is compromised in colitis. (a) The hepatic expression of enzymes involved in bile acid biosynthetic pathway. (b) Western blot analysis of CYP7A1 protein content in the liver. (c–e) Expression ofFxr,Fgf15andShpmRNAs in the distal ileum. (f) Expression ofFgfr4andβ-KlothomRNAs in the liver. (g) Immunohistochemistry staining and quantitative analysis of FXR protein content in the distal ileum (scale bar, 50 μm). (h) Immunohistochemistry staining and quantitative analysis of FGF15 protein content in the distal ileum (scale bar, 50 μm). Results of quantitative analysis values are expressed as mean±s.e.m. (n=6) and are plotted as fold change. *P<0.05, **P<0.01 versus normal control, Student’st-test. Figure 2: The intestinal FXR-FGF15 signalling is compromised in colitis. ( a ) The hepatic expression of enzymes involved in bile acid biosynthetic pathway. ( b ) Western blot analysis of CYP7A1 protein content in the liver. ( c – e ) Expression of Fxr , Fgf15 and Shp mRNAs in the distal ileum. ( f ) Expression of Fgfr4 and β-Klotho mRNAs in the liver. ( g ) Immunohistochemistry staining and quantitative analysis of FXR protein content in the distal ileum (scale bar, 50 μm). ( h ) Immunohistochemistry staining and quantitative analysis of FGF15 protein content in the distal ileum (scale bar, 50 μm). Results of quantitative analysis values are expressed as mean±s.e.m. ( n =6) and are plotted as fold change. * P <0.05, ** P <0.01 versus normal control, Student’s t -test. Full size image Intestinal FXR-FGF15 signalling is compromised in colitis As intestinal FXR-FGF15 signalling is the major determinant of hepatic CYP7A1 (refs 18 , 19 ), the possibility that intestinal FXR-FGF15 signalling is dysregulated in colitis was explored. No significant change was detected in the ileal Fxr mRNA ( Fig. 2c ) and protein content ( Fig. 2g ). However, the mRNA expression of FXR target genes, including Fgf15 and Shp ( Fig. 2d,e ), decreased markedly in colitis mice. Immunohistochemical staining also indicated a significantly decreased protein level of FGF15 in the ileum section ( Fig. 2h ). Of interest, the expression of Fgfr4 in the liver of colitis group was also decreased, while β-Klotho remained unchanged ( Fig. 2f ). These data indicate a decrease in the intestinal negative feedback pathway of bile acids synthesis in DSS-induced colitis mice. Glucuronidation of bile acids is facilitated in colitis FXR is a ligand-activated transcriptional factor and thus its activation is largely dependent on the intracellular level of its ligands. Colitis resulted in a significantly decreased level of multiple FXR ligands, including CDCA, DCA and CA, in the small intestine where they function to activate the FXR-FGF15 signalling ( Fig. 1f ). We thus reasoned that the decreased level of intracellular ligands of FXR in the small intestine might be one of the major mechanisms underlying the compromised FXR-FGF15 signalling in colitis. For this reason, the mechanisms responsible for the reduced intracellular levels of FXR ligands in the small intestine were investigated. The expression of transporters responsible for absorption of bile acids was measured in the distal ileum. Both apical and basal transporters, including Asbt , Ostα and Ostβ , and the intracellular bile acids binding protein Ibabp , remained largely unchanged ( Supplementary Fig. 3 ), suggesting that the reduction of intracellular FXR ligands is unlikely caused by bile acids malabsoprtion. In addition to cellular uptake capacity, metabolic elimination is another important determinant of the intracellular levels for both endogenous and exogenous agents. Quantitative analysis of bile acids species showed that the glucuronidation metabolites of bile acids were dramatically enhanced in both the faeces and urine ( Fig. 3a,b ). We thus checked whether the expression and activity of UGTs in the small intestine are elevated. The hepatic expression of Ugts has been previously been shown to play an important role in the metabolic elimination of bile acids [20] , [21] , [22] . However, very little is known about the role of intestinal UGTs in determining the homeostasis of bile acids. UGT1A3 and UGT2B4 were found to be the dominant UGT isoforms involved in the glucuronidation of bile acids in humans [20] , [23] ; however, the involvement of several other isoforms, including UGT1A4, UGT2B7, UGT2A1 and UGT2A2, has recently been reported [24] , [25] . These findings are in line with the general view about the largely overlapping property of UGTs in metabolism. Moreover, the exact UGT isoforms in the metabolism of bile acids in mice remains elusive. Thus, the major UGT isoforms expressed in the small intestine of mice [26] were determined. The mRNA levels for most of the Ugt isoforms, including Ugt1a6 , Ugt1a7 , Ugt2b24 and Ugt2b35 , were significantly upregulated in the small intestine of mice with DSS-induced colitis ( Fig. 3c ). Consistent with the mRNA data, the enzymatic activities for all the tested substrates in the small intestine of colitis mice were dramatically increased ( Fig.3d ). In particular, the intestinal enzymatic activity of CDCA glucuronidation was enhanced by fourfold ( Fig. 3d and Supplementary Table 1 ). This result strongly supports a facilitated metabolic elimination of potential FXR ligands from the intestinal epithelium and thus a significant reduction of intracellular levels of CDCA, CA and DCA, all of which are potent FXR ligands in mice. Moreover, human intestinal S9 fraction possessed a much stronger enzyme activity towards the glucuronidation of CDCA ( Supplementary Fig. 4 ), hinting to a more important role of intestinal UGTs in regulating the homeostasis of bile acids in humans. 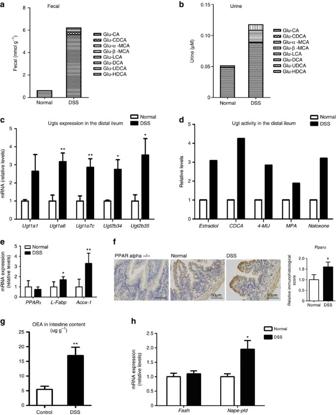Figure 3: Intestinal PPARα-UGTs axis is overactivated in colitis. (a,b) The quantitative analysis of glucuronidation metabolites of bile acids in faeces and urine. (c,d) Expression and enzyme activity of UGT1A1, UGT1A6, UGT1A7, UGT2B34 and UGT2B35. (e) Expression ofPparα,Acox1andL-FabpmRNAs in the small intestine. (f) Immunohistochemistry staining and quantitative analysis of PPARα protein content in the distal ileum (scale bar, 50 μm). (g) The concentration of OEA in the intestine contents of colitis mice, analysed by LC-MS. (h) The mRNA expression ofNape-pldandFaahin the small intestine. Results of mRNA expression are mean±s.e.m. of six mice. *P<0.05, **P<0.01 versus normal control, Student’st-test. Results of UGT activity were determined towards various substrates in pooled mice S9 (n=6); data are the means of triplicate determinations. Bile salts species were analysed by the UFLC-Triple-time of flight/MS analysis (n=6). Figure 3: Intestinal PPARα-UGTs axis is overactivated in colitis. ( a , b ) The quantitative analysis of glucuronidation metabolites of bile acids in faeces and urine. ( c , d ) Expression and enzyme activity of UGT1A1, UGT1A6, UGT1A7, UGT2B34 and UGT2B35. ( e ) Expression of Pparα , Acox1 and L-Fabp mRNAs in the small intestine. ( f ) Immunohistochemistry staining and quantitative analysis of PPARα protein content in the distal ileum (scale bar, 50 μm). ( g ) The concentration of OEA in the intestine contents of colitis mice, analysed by LC-MS. ( h ) The mRNA expression of Nape-pld and Faah in the small intestine. Results of mRNA expression are mean±s.e.m. of six mice. * P <0.05, ** P <0.01 versus normal control, Student’s t -test. Results of UGT activity were determined towards various substrates in pooled mice S9 ( n =6); data are the means of triplicate determinations. Bile salts species were analysed by the UFLC-Triple-time of flight/MS analysis ( n =6). Full size image Of interest, the mRNA levels and enzyme activity of some UGTs in the liver were also slightly increased ( Supplementary Fig. 5a,b ), consistent with the slightly increased glucuronidation products of bile acids in the urine of colitis mice. It was somewhat unexpected to find that the enzymatic expression and activity of multiple UGTs in the colon of colitis mice were also significantly enhanced ( Supplementary Fig. 5c,d ), in spite of the dramatic accumulation of multiple bile acids species in the colon tissues. Together, these results suggest that the expression and activity of UGTs and, in particular, in the GI tract are largely enhanced under the condition of colitis, facilitating the metabolic elimination of bile acids. PPARα underlies UGTs and bile acid disturbance in colitis Previous studies illustrated that PPARα is an important transcriptional factor in regulating the expression of various UGT enzymes [20] , [27] and can also regulate the homeostasis of bile acids by unclear mechanisms. Hence, we assume that PPARα may play a critical role in mediating the dysregulation of bile acids in colitis. The increased mRNA expression of Acox1 and L-Fabp suggests that the PPARα signalling pathway in the small intestine was activated in colitis mice ( Fig. 3e ). Although the ileal expression of Pparα mRNA was not significantly changed, immunohistochemical staining showed a slight increase in its protein expression ( Fig. 3e,f ). It was reported that oleylethanolamide (OEA) was a natural endogenous lipid that activates PPARα with high potency and exert anorectic actions [28] , [29] . Consequently, a prominent rationale is that the activation of PPARα pathway is dependent on the elevated concentration of its endogenous ligands. To this end, we investigated OEA levels by liquid chromatography–mass spectrometry and found a strongly enhanced level in the intestine contents of colitis mice ( Fig. 3g ). NAPE-PLD ( N -acyl phosphatidylethanolamine-selective phospholipase D) is responsible for the biosynthesis of OEA, while FAAH (fatty acid amide hydrolase) is involved in its degradation [30] . Here, the upregulated expression of Nape-pld mRNA and the unchanged expression of Faah mRNA ( Fig. 3h ) suggest that the increased level of OEA in colitis mice is likely due to the enhanced biosynthesis. The increased OEA biosynthesis, upregulation of PPARα typical target genes, together with the upregulated expression of Ugts suggest an activated PPARα-UGTs axis in the intestine of colitis mice. To ascertain whether the PPARα activation can regulate intestinal FXR-FGF15 signalling and the bile acid homeostasis, normal mice were administered with the PPARα agonist Wy-14643. Wy-14643 treatment for 1 week significantly upregulated the mRNAs of typical PPARα target genes Acox1 and L-Fabp in the small intestine ( Supplementary Fig. 6a–c ) and resulted in a robust enhancement of the intestinal expression of multiple Ugts ( Fig. 4b ). In particular, the enzymatic activity towards the glucuronidation of CDCA was enhanced 21-fold by Wy-14643 treatment ( Fig. 4a ). These results strongly suggest that the intestinal PPARα plays a pivotal role in regulating the glucuronidation of bile acids. Next, we determined whether the activation of intestinal PPARα-UGTs axis could regulate the intestinal FXR-FGF15 signalling and, thereafter, bile acids homeostasis. Wy-14643 treatment significantly suppressed ileum expression of Fgf15 ( Fig. 4c ) and increased the hepatic expression of Cyp7a1 ( Fig. 4d,e ), while the intestinal Fxr expression was not significantly affected ( Fig. 4c ). Notably, the intestinal FXR-FGF15 signalling regulated by Wy-14643 was quite similar to that observed in DSS-induced colitis. Thus, we next asked whether the PPARα activation by Wy-14643 could mimic the alternation of bile acids distribution pattern observed in colitis. The results showed that Wy-14643 treatment reduced levels of bile acids in the small intestine ( Fig. 4f ) but increased the bile acids levels in the colon and faeces ( Supplementary Fig. 7 ); moreover, the faecal glucuronides of most bile acid species were much higher in the mice with Wy-14643 treatment than that in the control ( Supplementary Fig. 6d ). This profile largely mimics that observed under the condition of colitis, except that the colonic accumulation of some bile acids species is less evident than those in colitis. Together, these findings strongly support an important role of intestinal PPARα activation in compromising the intestinal FXR-FGF15 feedback signalling that leads to a continuous upregulation of CYP7A1 and the enhanced de-novo bile acids synthesis. 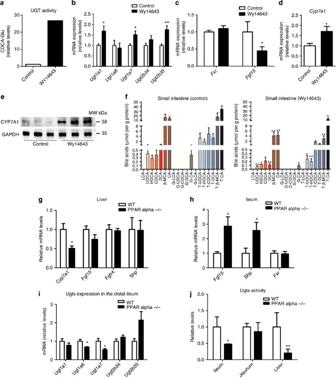Figure 4: PPARα controls intestinal FXR-FGF15 and bile acid homeostasis. (a–f) The mice were treated with Wy-14643 (50 mg kg−1, i.g., once a day) for 1 week. Results are mean±s.e.m. of eight mice. *P<0.05, **P<0.01 versus control, Student’st-test. (a) The enzymatic activity of UGT isozymes towards the gluronidation of CDCA. The mice S9 in the distal ileum were a pool of eight individuals. (b) The mRNA expression ofUgt1a1,Ugt1a6,Ugt1a7,Ugt2b34andUgt2b35. (c) The ileum expression ofFxrandFgf15in control and Wy-14643-treated mice. (d,e) The hepatic expression and protein content of CYP7A1 in control and WY-14643-treated mice. (f) Small intestinal bile acid profiles of control and Wy-14643-treated mice using UFLC-triple-time of flight analysis. (g–j) Comparative study inPpara-null and WT mice; results of quantitative analysis values are expressed as mean±s.e.m. (n=6) and are plotted as fold change. *P<0.05, **P<0.01 versus WT, Student’st-test. (g) The hepatic expression ofCyp7a1,Fgf15,Fgfr4andShpin WT andPpara-null (Pparα−/−) mice. (h) Expression ofFgf15,ShpandFxrmRNAs in the ileum. (i,j) The mRNA expression and activity ofUgtsin control andPpara-null mice. Figure 4: PPARα controls intestinal FXR-FGF15 and bile acid homeostasis. ( a – f ) The mice were treated with Wy-14643 (50 mg kg −1 , i.g., once a day) for 1 week. Results are mean±s.e.m. of eight mice. * P <0.05, ** P <0.01 versus control, Student’s t -test. ( a ) The enzymatic activity of UGT isozymes towards the gluronidation of CDCA. The mice S9 in the distal ileum were a pool of eight individuals. ( b ) The mRNA expression of Ugt1a1 , Ugt1a6 , Ugt1a7 , Ugt2b34 and Ugt2b35 . ( c ) The ileum expression of Fxr and Fgf15 in control and Wy-14643-treated mice. ( d , e ) The hepatic expression and protein content of CYP7A1 in control and WY-14643-treated mice. ( f ) Small intestinal bile acid profiles of control and Wy-14643-treated mice using UFLC-triple-time of flight analysis. ( g – j ) Comparative study in Ppara -null and WT mice; results of quantitative analysis values are expressed as mean±s.e.m. ( n =6) and are plotted as fold change. * P <0.05, ** P <0.01 versus WT, Student’s t -test. ( g ) The hepatic expression of Cyp7a1 , Fgf15 , Fgfr4 and Shp in WT and Ppara -null ( Pparα −/− ) mice. ( h ) Expression of Fgf15 , Shp and Fxr mRNAs in the ileum. ( i , j ) The mRNA expression and activity of Ugts in control and Ppara -null mice. Full size image To further validate the role of PPARα in regulating intestinal FXR-FGF15 signalling, a comparative study between wild-type (WT) mice and Pparα -null mice was performed ( Supplementary Fig. 8a ). In agreement with a recent study [31] , hepatic expression of Cyp7a1 mRNA in Ppara -null mice was much lower than that in WT mice ( Fig. 4g ). The downregulation of hepatic Cyp7a1 in Pparα -null mice is at least partially due to the increased intestinal upregulation of Fgf15 ( Fig. 4h ). In support of a role for PPARα in regulating intestinal UGTs, the intestinal expression of several Ugt genes was significantly lower than in WT mice ( Fig. 4i ). The enzymatic activity towards the glucuronidation of CDCA in the intestinal S9 fraction of Ppara -null mice was lower than that in WT mice ( Fig. 4j ). Moreover, the faecal glucuronides of most bile acid species were much lower in the Ppara -null mice than that in WT mice ( Supplementary Fig. 8b ). PPARα-UGTs axis controls FXR-FGF19 signalling in enterocytes To further validate the role of PPARα-UGTs axis in the regulation of bile acids homeostasis, a cellular pharmacokinetic study of CDCA and its association with FXR-FGF15 (FGF19 in humans) signalling was carried out. In a rat intestinal epithelial cell line IEC-6, treatment with Wy-14643 significantly increased the production of CDCA glucuronide ( Supplementary Fig. 9a ). Moreover, the intracellular exposure level of CDCA was decreased by Wy-14643 treatment, which was closely associated with a significant reduction in activating Fxr-Fgf15 ( R 2 =0.8621, P =0.0003, for test of close fit) (Supplementary Fig. 9b–d). The experiments conducted in primary murine intestinal epithelial cells (PMIECs) further validated these findings. Both OEA and Wy-14643 treatment significantly promoted the metabolic elimination of CDCA and CA in PMIECs, as judged by decreased intracellular concentrations of CDCA and CA, and increased glucuronides of them ( Fig. 5a,b,d,e ). Consistently, the expression of FXR target genes Fgf15 and Shp was markedly reduced on OEA and Wy-14643 treatment ( Fig. 5c,f ), indicating a repressed FXR activation as a result of PPARα activation. 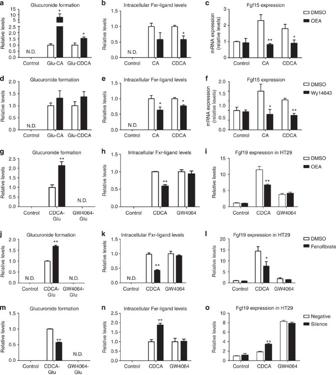Figure 5: PPARα-UGTs axis controls FXR-FGF15 signalling in enterocytes. (a–f) PMIECs were incubated with 50 μM of CA or CDCA in the absence or presence of PAPRα agonists. (a–c) The relative levels of glucuronidation metabolites in the media and the intracellular concentration of FXR ligands and the expression ofFgf15in PMIECs under treatment with OEA. (d–f) The relative levels of glucuronidation metabolites in the media and the intracellular concentration of FXR ligands, and the expression ofFgf15in PMIECs under the treatment of Wy-14643. (g–i) The relative levels of glucuronidation metabolites in the media and intracellular concentrations of FXR ligands, and the expression ofFGF19in HT29 cells under the treatment of OEA. (j–l) The relative levels of glucuronidation metabolites in the media and the intracellular concentration of FXR ligands, and the expression ofFGF19in HT29 cells under the treatment of fenofibrate. (m–o) The relative levels of glucuronidation metabolites in the media and intracellular concentration of FXR ligands, and the expression ofFGF19of control and UGT1A3 siRNA-transfected HT29 cells. Data are the mean±s.e.m. of three independent experiments and are plotted as fold change. *P<0.05, **P<0.01 versus control, Student’st-test. Figure 5: PPARα-UGTs axis controls FXR-FGF15 signalling in enterocytes. ( a – f ) PMIECs were incubated with 50 μM of CA or CDCA in the absence or presence of PAPRα agonists. ( a – c ) The relative levels of glucuronidation metabolites in the media and the intracellular concentration of FXR ligands and the expression of Fgf15 in PMIECs under treatment with OEA. ( d – f ) The relative levels of glucuronidation metabolites in the media and the intracellular concentration of FXR ligands, and the expression of Fgf15 in PMIECs under the treatment of Wy-14643. ( g – i ) The relative levels of glucuronidation metabolites in the media and intracellular concentrations of FXR ligands, and the expression of FGF19 in HT29 cells under the treatment of OEA. ( j – l ) The relative levels of glucuronidation metabolites in the media and the intracellular concentration of FXR ligands, and the expression of FGF19 in HT29 cells under the treatment of fenofibrate. ( m – o ) The relative levels of glucuronidation metabolites in the media and intracellular concentration of FXR ligands, and the expression of FGF19 of control and UGT1A3 siRNA-transfected HT29 cells. Data are the mean±s.e.m. of three independent experiments and are plotted as fold change. * P <0.05, ** P <0.01 versus control, Student’s t -test. Full size image To provide a translational link to humans, this study was extended to HT29 cells by using OEA and fenofibrate (a specific human PPARα agonist) treatment. The cellular kinetic profiles clearly indicated that the activation of PPARα by OEA and fenofibrate dramatically decreased intracellular level of CDCA, while small interfering RNA (siRNA) silencing of UGT1A3 significantly increased CDCA levels ( Supplementary Fig. 10a–d ). In addition, treatment of HT29 cells with OEA markedly promoted the production of CDCA glucuronide and reduced the intracellular level of CDCA, leading to decreased expression of FGF19 ( Fig. 5g–i ). The results obtained from fenofibrate were quite similar to that observed on OEA treatment ( Fig. 5j–l ). Moreover, the results from the siRNA silencing of PPARα study confirmed that fenofibrate elicits its effects in a PPARα-dependent manner ( Supplementary Fig. 10e–g ). The siRNA silencing of UGT1A3 drastically increased the intracellular levels of CDCA and reduced the production of CDCA glucuronide, translating to a twofold enhancement of FGF19 expression ( Fig. 5m–o ). Interestingly, PPARα activation and Ugt1a3 knockdown could not influence the intracellular level of GW4064, a typical FXR agonist, as well as the activation of the FXR-FGF19 signalling pathway ( Fig. 5g–o ), because GW4064 is not a substrate of UGTs and thus is not glucuronidated in HT29 cells. Together, results from the in vitro cellular study provide direct evidence supporting a pivotal role for PPARα and UGTs in determining the intestinal FXR-FGF15 signalling via controlling the intracellular disposition of FXR ligands. Results obtained from the study in HT29 cells suggest that disruption of the PPARα-UGTs axis can also compromise the intestinal FXR-FGF19 signalling in humans. To develop a translational link to humans, possible dysregulation of PPARα-UGTs and FXR-FGF19 signalling in the colon biopsies from IBD patients was analysed. In line with data obtained from the DSS-induced colitis mice, the PPARα target genes, including ACOX1 and multiple UGTs , in particular the UGT1A3 , were significantly higher, while expression of the FXR target genes, including FGF19 and SHP , were significantly lower than that in the healthy control samples ( Supplementary Fig. 11a–c ). These results indicate that PPARα-UGTs signalling is overactivated and may repress the FXR-FGF19 signalling in IBD patients. PPARα-FGF15 signalling controls DSS-induced colitis The present results indicated that the PPARα-FGF15 signalling has a pivotal role in determining bile acid homeostasis under both physiological conditions and in DSS-induced colitis. To determine whether dysregulation of PPARα-FGF15 signalling is involved in the pathological development of DSS-induced colitis, mice were treated with PPARα agonist Wy-14643 alone or together with DSS. Although Wy-14643 alone did not induce any inflammatory change in the colon, it markedly enhanced DSS-induced colitis. In a preliminary study, we found that Wy-14643 together with a relatively low dose of DSS at 2% resulted in a high mortality rate and most of the mice could not survive through the three cycles of DSS treatment. Thus, we designed an experimental protocol of 7 days DSS treatment with 3 days washout to determine the influence of PPARα activation in DSS-induced colitis. By use of this protocol, DSS alone induced a relatively minor extent of inflammatory damage and less evident upregulation of UGTs ( Supplementary Fig. 12c ), as compared with the chronic DSS-induced colitis ( Fig. 3c ). Wy-14643 co-treatment with DSS resulted in a more dramatic decrease in body weight and colon length ( Fig. 6a,b ), more severe inflammatory damage ( Fig. 6c ) and higher extent of imbalance between proinflammatory and anti-inflammatory cytokines ( Supplementary Fig. 12a ), when compared with DSS treatment alone. Wy-14643 treatment significantly upregulated the expression of Pparα and its target genes in the ileum, including Acox-1 , L-Fabp and multiple Ugt isoform genes ( Supplementary Fig. 12b,c ). Consistently, the ileum expression of FXR target genes Fgf15 and Shp , and hepatic expression of Fgfr4 and Shp were further decreased ( Fig. 6d,e ), leading to more upregulated expression of hepatic Cyp7a1 and increased bile acid pool size in the Wy-14643 and DSS co-treated mice ( Fig. 6e,f ). 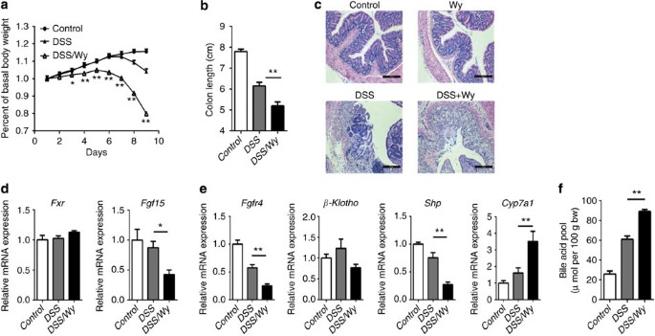Figure 6: Wy-14643 exacerbates DSS-induced colitis. (a) Body weight. (b) Colon length. (c) Histological assessment (scale bar, 100 μm). (d) Ileum expression ofFxrandFgf15mRNAs. (e) Hepatic expression ofFgfr4,β-Klotho,ShpandCyp7a1mRNAs. (f) Bile acid pool analysis. Results of quantitative analysis values are expressed as mean±s.e.m. (n=6) and are plotted as fold change. *P<0.05, **P<0.01 versus DSS, Student’st-test. Figure 6: Wy-14643 exacerbates DSS-induced colitis. ( a ) Body weight. ( b ) Colon length. ( c ) Histological assessment (scale bar, 100 μm). ( d ) Ileum expression of Fxr and Fgf15 mRNAs. ( e ) Hepatic expression of Fgfr4 , β-Klotho , Shp and Cyp7a1 mRNAs. ( f ) Bile acid pool analysis. Results of quantitative analysis values are expressed as mean±s.e.m. ( n =6) and are plotted as fold change. * P <0.05, ** P <0.01 versus DSS, Student’s t -test. Full size image To further validate the role of PPARα in colitis, a comparative study of DSS-induced colitis was performed in WT and Ppara -null mice. Ppara -null mice were less susceptible to chronic DSS-induced colitis, as judged by less decrease in body weight, longer colon length and reduced inflammatory tissue damage, when compared with WT mice ( Fig. 7a–c ). The ileum expression of PPARα target gene L-Fabp and multiple Ugt isoform genes, including Ugt1a1 , Ugt1a6 and Ugt1a7 in the Pparα -null mice, was significantly lower than that in the WT littermates ( Fig. 7d,e ). Consequently, the ileum expression of FXR target genes Fgf15 and Shp was significantly higher, while the hepatic expression of Cyp7a1 was significantly lower in the Ppara -null mice than that in the WT littermates ( Fig. 7f,g ). 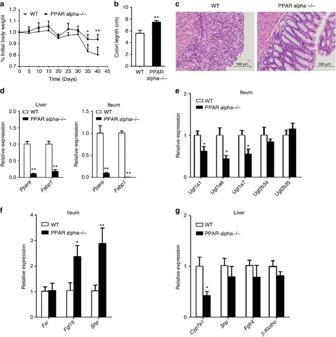Figure 7:Pparα-null mice are less susceptible to DSS-induced colitis. (a) Body weight. (b) Colon length. (c) Haematoxylin and eosin staining of colon tissues (scale bar, 100 μm). (d) The mRNA expression ofPparαandL-Fabpin the ileum and liver of WT control andPparα-null (Pparα−/−) mice. (e) The mRNA expression ofUgtsin WT andPparα−/− mice. (f) The mRNA expression ofFgf15,ShpandFxrin the ileum. (g) The hepatic expression ofCyp7a1,β-Klotho,Fgfr4andShpin WT andPparα−/− mice. Results of quantitative analysis values are expressed as mean±s.e.m. (n=6) and are plotted as fold change. *P<0.05, **P<0.01 versus WT, Student’st-test. Figure 7: Pparα -null mice are less susceptible to DSS-induced colitis. ( a ) Body weight. ( b ) Colon length. ( c ) Haematoxylin and eosin staining of colon tissues (scale bar, 100 μm). ( d ) The mRNA expression of Pparα and L-Fabp in the ileum and liver of WT control and Pparα -null ( Pparα −/−) mice. ( e ) The mRNA expression of Ugts in WT and Pparα −/− mice. ( f ) The mRNA expression of Fgf15 , Shp and Fxr in the ileum. ( g ) The hepatic expression of Cyp7a1 , β-Klotho , Fgfr4 and Shp in WT and Pparα −/− mice. Results of quantitative analysis values are expressed as mean±s.e.m. ( n =6) and are plotted as fold change. * P <0.05, ** P <0.01 versus WT, Student’s t -test. Full size image As the reduced ileum secretion of FGF15 is an important determinant in causing dysregulation of bile acids in DSS-induced colitis, the possibility that FGF15 supplementation could ameliorate DSS-induced colitis and restore bile acid homeostasis was investigated. As it was previously reported that recombinant human FGF19 is effective in regulating bile acid homeostasis in mice [32] , DSS-induced colitis mice were treated with recombinant human FGF19 at a dose of 25 μg kg −1 intraperitoneally. Chronic treatment of FGF19 markedly attenuated DSS-induced colitis, as revealed by a significant increase in the ability to regain weight, longer colon length and improved inflammatory tissue damage ( Fig. 8a–c ). Moreover, FGF19 treatment significantly restored hepatic expression of Fgfr4 and Shp , and in particular, the hepatic expression of Cyp7a1 , and the bile acid pool size returned to normal levels ( Fig. 8d–g ). Together, these results suggest that reduced secretion of FGF15 is an important factor in facilitating pathological development of DSS-induced colitis and that the chronic FGF19 treatment at a low dose may be a promising strategy for therapy of colitis. 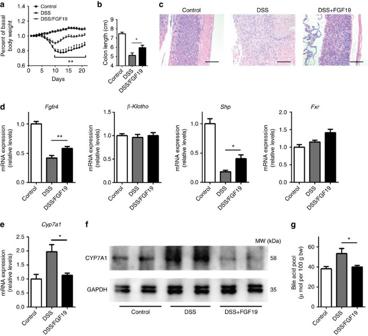Figure 8: FGF19 treatment protects against DSS-induced colitis in mice. DSS-induced chronic colitis mice were treated with recombinant FGF19 at a dose of 25 μg kg−1per day for the first 14 days per DSS cycle. (a) Body weight recorded during the first DSS cycle. (b) Colon length. (c) Haematoxylin and eosin staining of colon tissues (scale bar, 100 μm). (d) HepaticFgfr4,β-klotho,ShpandFxrmRNA expression. (e) HepaticCyp7a1mRNA expression. (f) Hepatic levels of CYP7A1 protein. (g) Bile acid pool analysis. Results of quantitative analysis values are mean±s.e.m. of eight mice. *P<0.05, **P<0.01 versus DSS, Student’st-test. Figure 8: FGF19 treatment protects against DSS-induced colitis in mice. DSS-induced chronic colitis mice were treated with recombinant FGF19 at a dose of 25 μg kg −1 per day for the first 14 days per DSS cycle. ( a ) Body weight recorded during the first DSS cycle. ( b ) Colon length. ( c ) Haematoxylin and eosin staining of colon tissues (scale bar, 100 μm). ( d ) Hepatic Fgfr4 , β-klotho , Shp and Fxr mRNA expression. ( e ) Hepatic Cyp7a1 mRNA expression. ( f ) Hepatic levels of CYP7A1 protein. ( g ) Bile acid pool analysis. Results of quantitative analysis values are mean±s.e.m. of eight mice. * P <0.05, ** P <0.01 versus DSS, Student’s t -test. Full size image The current study demonstrated that chronic DSS-induced colitis activates intestinal PPARα-UGTs axis promoting the metabolic elimination of bile acids, endogenous ligands of FXR, in the small intestine. The reduced intracellular level of endogenous FXR ligands results in a repressed activation of intestinal FXR-FGF15 feedback signalling that leads to the upregulation of hepatic CYP7A1 and thereby increasing de novo synthesis of bile acids under conditions of DSS-induced colitis. Our results indicate that the overactivation of the PPARα-UGT axis and consequently the compromised intestinal FXR-FGF15 signalling are key determinants in the pathological development of colitis in the DSS-induced model. Increased faecal excretion of bile acids is a well-defined pattern in IBD; however, the potential altered disposition of bile acids in other compartments in IBD is less known and controversial in previous studies [33] , [34] . Increased faecal excretion but decreased serum levels of bile acids were observed in experimental colitis mice, which conformed to earlier observations in both experimental colitis and IBD patients [35] , [36] . The levels of bile acids accumulated in the inflamed colon tissues were found dramatically increased, supporting a potential role for toxic bile acids in potentiating the pathological development of colitis. Although the bile acid pool size increased, it was of interest to note that multiple unconjugated bile acids significantly decreased in the small intestine. The decreased intracellular levels of multiple FXR ligands, including CDCA, CA and DCA, in the ileum represent a major mechanism underlying the repressed FXR-FGF15 feedback signalling pathway in colitis. Moreover, the hepatic expression of Fgfr4 was reduced in colitis, which may be related to the reduced FGF15 levels in view that the FGF19 treatment could significantly restore the hepatic expression of Fgfr4 . The reduced circulating FGF15 levels and decreased hepatic expression of its receptor Fgfr4 may work together to upregulate CYP7A1. It was of interest to note that the intracellular accumulation of TβMCA, a recently identified endogenous FXR antagonist [37] , [38] , in the ileum is significantly increased in colitis mice. Thus, the possibility cannot be excluded that the increased level of FXR antagonist TβMCA, in addition to a decrease in FXR agonists, may also contribute to compromised ileal FXR-FGF15 signalling in colitis mice. Nevertheless, these findings suggest a facilitated faecal elimination and an increased hepatic de novo synthesis of bile acids in DSS-induced colitis. Such a dysregulation of bile acids in DSS-induced colitis is quite similar to that observed from the use of bile acids sequestrant, which promotes the faecal elimination of bile acids and upregulates the hepatic expression of Cyp7a1 . Of particular interest, a recent study suggested a specific enrichment of bile acids in the colon with colestilan treatment [39] . It seems that the facilitated faecal elimination of bile acids may be able to promote the delivery of bile acids to the distal part of the gut. The inflamed colon tissues characterized with damaged epithelium are thus readily to enrich bile acids species. As the faecal excretion of uncojungated bile acids is even higher in colitis mice than that in the normal control, the reduced intracellular uncojungated bile acids in the small intestine may not be explained by the reduced deconjugation activity in the colitis mice. Instead, these results strongly indicate that the glucuronidation of bile acids in colitis mice is drastically increased, which may explain the reduced intracellular levels of uncojungated bile acids. Unlike taurine- and glycine-conjugated bile acids, glucuronidated bile acids cannot be reabsorbed and may represent an important detoxification mechanism under the condition of abnormal bile acids accumulation [21] . Previous studies suggested that the hepatic glucuronidation of bile acids may be part of a negative feedback mechanism by which bile acids limit their biological activity and control their intracellular level to avoid a pathophysiological accumulation [23] , [40] . The present data suggest that the intestinal glucuronidation of bile acids is also an important factor in maintaining the bile acid homeostasis via controlling the intracellular levels of endogenous FXR ligands and consequently the ileal FXR-FGF15 signalling. Although it remains still a concern about the exact UGT isoforms involved in the glucuronidation of bile acids in mice, it is reasonable to speculate that multiple UGT isoforms may be involved, considering that multiple UGT isoforms, including UGT1A3, UGT2B4, UGT2B7, UGT2A1 and UGT2A2, were found responsible for bile acid glucuronidation in human beings [20] , [24] , [25] . Previous studies about the effect of PPARα activation in regulating CYP7A1 and bile acids homeostasis are controversial. Some studies reported that activation of PPARα by fibrates could repress the expression of Cyp7a1 (refs 41 , 42 ), which was presumed to be a potential mechanism underlying the side effects of fibrates in causing gall stones in humans. However, other studies indicated that the activation of PPARα by endogenous agonist, such as fatty acid metabolites, could promote Cyp7a1 transcriptional activity [43] and that the PPARα-specific agonist Wy-14643 increased the bile acid synthesis in mice [44] . However, none of the previous studies considered the potential influence of PPARα activation in regulating CYP7A1 via the intestinal FXR-FGF15 signalling. The current finding that increased OEA, an endogenous PPARα ligand, and the resultant upregulation of typical PPARα target genes and genes encoding some of the UGTs in the small intestine, indicate an activated PPARα-UGTs axis in colitis mice. Oral administration of the PPARα agonist Wy-14643 largely mimicked the characteristic patterns observed in colitis, including the enhanced UGT expression and activity, repressed intestinal FXR-FGF15 signalling, upregulated hepatic CYP7A1 expression and even the compartmental disposition patterns of bile acids. Moreover, the intestinal FXR-FGF15 feedback signalling was found significantly promoted in the Pparα -null mice. In PMIECs, PPARα activation by Wy-14643 or OEA led to repressed FXR-FGF15 signalling activated by CDCA or CA, an effect that was dependent on the expression and activity of UGTs. Notably, the activation of PPARα by OEA or fenofibrate in the HT29 cell lines led to quite similar findings to that observed in the rodent intestinal cell model. The analysis of colon biopsies further reveals that activation of the PPARα-UGTs axis and repression of FXR-FGF19 signalling also occurs in IBD patients. Moreover, chronic treatment with fenofibrate for three months markedly reduced the serum levels of FGF19 (ref. 45 ), supporting an important role of PPARα activation in regulating FXR-FGF19 signalling in humans. Together, these results provide a translational link of the findings from the DSS-induced colitis mice to the pathological development of IBD in humans. Several previous reports suggest a protective effect of PPARα activation against the pathological development of experimental colitis [46] , [47] , [48] , [49] , which are contradictory to the present findings. Herein, a comprehensive evidence is provided that the intestinal PPARα is already overactivated in the chronic DSS-induced colitis model, and that the treatment with PPARα agonist could markedly promote, whereas the knockout of PPARα could significantly retard, the pathological development of DSS-induced colitis. Moreover, the chronic treatment with recombinant FGF19 could significantly attenuate DSS-induced colitis. The discrepancy between the present results and the previous reports may be explained by the use of different animal models and experimental protocols. Notably, previous studies were performed either in acute colitis animal models or in the interleukin-10-deficient mice that spontaneously develop colitis. The protective effects of PPARα activation observed with these mouse models may be explained by the anti-inflammatory effects of PPARα activation. In contrast, the present study showed that prolonged activation of PPARα in the DSS-induced chronic colitis model may actually aggravate the pathological development of colitis via disrupting bile acid homeostasis. Previous studies revealed that in a 2,4,6-trinitrobenzenesulfonic acid-induced acute colitis model, most of the UGTs were downregulated [50] . Moreover, the present study revealed that the upregulation of UGTs in the acute DSS colitis-treated mice is less evident than that in the chronic DSS models. These results suggest that the PPARα-UGTs dysregulation patterns may vary between acute and chronic colitis animal models. However, even in the acute DSS-induced colitis, the prolonged treatment (10 days) with Wy-14643 drastically exacerbated the pathological development of colitis ( Fig. 6a–f ). Together, our results support a pivotal role of prolonged PPARα activation and the resultant bile acids dysregulation in the pathological development of chronic DSS-induced colitis. In summary, the current study indicates that the intestinal PPARα-UGT axis plays a pivotal role in regulating FXR-FGF15 (FGF19) signalling and bile acid homeostasis via controlling the intracellular levels of FXR ligands. Under conditions of DSS-induced chronic colitis, the prolonged activation of intestinal PPARα-UGT axis promotes the intracellular metabolic elimination of endogenous FXR ligands in the small intestine, which decouples the intestinal FXR-FGF15 feedback signalling from the hepatic CYP7A1 expression and bile acids de novo synthesis ( Fig. 9 ). Results collected from the present study suggest that restoration of OEA-PPARα-UGT axis and FXR-FGF15 signalling may be of benefits to restore bile acid homeostasis in the colitis model and thus retard pathological development of colitis. Taken together, these results suggest that the regulation of PPARα–UGT axis and the supplementation of recombinant FGF19 may represent promising strategy for the therapy of colitis. 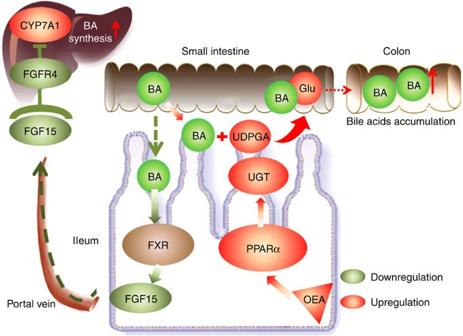Figure 9: PPARα-UGTs axis regulates bile acid homeostasis in colitis. In the ileum, the activation of PPARα due to the increased levels of OEA upregulates Ugts, which facilitate the metabolic elimination of bile acid endogenous ligands for FXR. The reduced intracellular level of FXR ligands in the ileum compromises FXR-FGF19/15 signalling and represses the hepatic expression of CYP7A1, promotingde-novosynthesis of bile acids. The PPARα-UGTs axis is functionally overactivated in colitis and represents a major mechanism in bile acids homeostasis disruption. The increased delivery of bile acids to the inflamed colon where the mucosa integrity is damaged by inflammation results in an abnormal accumulation of toxic bile acids and thereby facilitates the pathological development of colitis. Figure 9: PPARα-UGTs axis regulates bile acid homeostasis in colitis. In the ileum, the activation of PPARα due to the increased levels of OEA upregulates Ugts, which facilitate the metabolic elimination of bile acid endogenous ligands for FXR. The reduced intracellular level of FXR ligands in the ileum compromises FXR-FGF19/15 signalling and represses the hepatic expression of CYP7A1, promoting de-novo synthesis of bile acids. The PPARα-UGTs axis is functionally overactivated in colitis and represents a major mechanism in bile acids homeostasis disruption. The increased delivery of bile acids to the inflamed colon where the mucosa integrity is damaged by inflammation results in an abnormal accumulation of toxic bile acids and thereby facilitates the pathological development of colitis. Full size image Materials OEA was purchased from Santa Cruz Biotechnology (Santa Cruz, CA); DSS (molecular weight=36,000–50,000 kDa) was obtained from MP Biochemical (Santa Ana, CA). MPA O -glucuronide and naloxone 3-β-D-glucuronide were obtained from Toronto Research Chemicals Inc. (ON, Canada). β-MCA, UDCA, HDCA, G-LCA, G-UDCA, G-DCA, T-β-MCA, T-UDCA, T-HDCA and T-LCA were purchased from Steraloids Inc. (Newport, RI). α-MCA, CA, DCA, CDCA, lithocholic acid (LCA), G-CDCA, G-CA, T-CDCA, T-DCA, T-CA, dehydrocholic acid and propranolol were purchased from Sigma-Aldrich (St Louis, MO). The anti-UGT1A, anti-FXR, anti-FGF15 and anti-CYP7A1 antibodies were purchased from Santa Cruz Biotechnology. The anti-PPARα antibody was from Abcam (Cambridge, UK). The anti-glyceraldehyde-3-phosphate dehydrogenase (GAPDH) antibody was purchased from SunShine Biotechnology (Nanjing, China). The secondary antibodies and recombinant human FGF19 was obtained from Bioworld Technology (St Louis Park, MN). Other reagents, unless mentioned, were obtained from Sigma-Aldrich. RNA extracts of colon biopsies from 8 healthy humans and 13 ulcerative colitis and Crohn’s disease patients were previously described [51] . The ulcerative colitis and Crohn’s disease samples were collected from consented patients and approved by the University of Michigan IRB committee (approval number HUM00042210). Animals and treatments Specific pathogen free male C57BL/6 mice (8 weeks old, 20 g) were obtained from Academy of Military Medical Sciences, China. Animals were housed in an air-conditioned room (25 °C) under a 12-h light/dark cycle for 1 week before experiments and allowed water and standard chow ad libitum . Mice were randomly classified into different groups according to body weights in all the experiments. The animal studies were approved by the Animal Ethics Committee of China Pharmaceutical University and have been carried out in accordance with the Declaration of Helsinki. Pparα -null mice and WT mice on a C57BL/6N genetic background were raised and maintained in the National Cancer Institute; handling was in accordance with an animal study protocol approved by the National Cancer Institute Animal Care and Use Committee. Colitis was induced using the method described before with little modification [52] . In brief, colitis was induced by administration of 2.5% (w/v) DSS in drinking water for 7 days and a 14-day washout with drinking water for 3 cycles. Faecal and urine excretion of bile acid was determined in stools collected over 24 h in metabolic cages. Mice were killed at the indicated time points after induction of experimental colitis. Blood was collected from the post-ocular vein. Liver, small intestine, colon and intestine content were harvested and the small intestine was divided into three equal segments in ascending order. To determine the total bile acid content, tissues were removed from 4-h-fasted mice. All tissues for bile acid and RNA analysis were snap frozen in liquid nitrogen and stored in −80 °C until further processed. For the PPARα activation study, male, 8-week-old mice were administered Wy-14643 (50 mg kg −1 per day) or vehicle (0.5% CMC-Na) by intragastric gavage at 0800, h each day for 1 week. Mice were killed 24 h after the last dose, and the organs were collected and stored at −80 °C until analysis. To determine the role of PPARα activation in the pathological development of colitis, mice were randomly divided into three groups, including Wy-14643 group (Wy-14643 containing diet, ~50 mg kg −1 per day), DSS group (2% in drinking water) and DSS+Wy-14643 group. DSS were treated for 7 days and then replaced with drinking water for 3 days. The mice were killed on the day 10 for experimental determinations. To determine the influence of FGF19 in DSS-induced colitis, male, 8-week-old mice were treated with or without 25 μg kg −1 of FGF19 intraperitoneally (at 1800, h, once a day on the first 14 days of each DSS cycle) throughout the three cycles of DSS treatment (2% DSS in drinking water for 7 days, a 14-day washout with drinking water in each cycle). Cell culture and treatment The rat intestinal epithelial cell line IEC-6 was obtained from the goldamethyst Pharm and Bio-tech Co. Ltd (Beijing, China). Human colon carcinoma cell line HT29 was obtained from American Type Culture Collection (Manassas, USA). IEC-6 cells were grown in DMEM (GIBCO, Gland Island, New York) supplemented with 0.1 U ml −1 bovine insulin and 1 × MEM noniessential amino acids (Invitrogen, Carlsbad, CA, USA). HT-29 cells were cultured in McCoy’s 5A medium (GIBCO). The PMIECs were isolated using chelation method as previously described [53] . Briefly, ileum was dissected from C57BL/6 mice and thoroughly washed with sterilized PBS. Ileum was cut into 1-mm pieces followed by incubation in the chelation buffer at room temperature that allowed the isolation of single epithelial cells. The isolated epithelial cells were suspended in advanced DMEM/F12 (Invitrogen) containing recombinant human epidermal growth factor 5 ng ml −1 , insulin 5 μg ml −1 , transferrin 5 μg ml −1 , epinephrine 1.0 μM, hydrocortisone 5 μg ml −1 , heparin sulphate 0.75 U ml −1 and ascorbic acid 50 μg ml −1 . All media were supplemented with 10 U ml −1 penicillin, 10 μg ml −1 streptomycin and 10% FCS. HT29 cells were maintained in culture for 7 days to allow differentiation into mature enterocyte-like cells. CDCA (50 μM), CA (50 μM) or GW4064 (5 μM) were used as natural or synthetic FXR agonists. OEA (50 μM), Wy-14643 (75 μM) and fenofibrate (50 μM) were used as murine or human-specific PPARα agonists. HT29 cells were transfected with control siRNA or siRNA targeting UGT1A3 (Invitrogen) using RNAiMAX transfection reagent (Invitrogen) according to the manufacturer’s instruction. Two days later, the cells were harvested for western blot analysis to confirm the efficiency of siRNA knockdown. For glucuronidation assays, the cells were treated with OEA, Wy-14643 or fenofibrate for 24 h and subsequently incubated in the presence of CA, CDCA or GW4064 for another 24 h. Media was then recovered for subsequent determination of metabolite. Cells were lysed by three freeze–thaw cycles for CA or CDCA determination. The quantification of CA, CDCA and glucuronidation metabolites were performed by liquid chromatography coupled to tandem mass spectrometry (LC-MS/MS) [20] , [54] . The chromatographic system consisted of a Shimadzu (Kyoto, Japan) LC system performed on API4000 (AB Sciex, Foster City, CA, USA). Analytes were separated with a ZOEBAX Eclipse Plus C18 column (2.1 × 150 mm, 3.5 μm) (Agilent Technologies, USA). The mobile phase consisted of solvent A 2.6 mmol l −1 ammonium acetate in water and solvent B acetonitrile. A gradient elution of the mobile phase was performed: initial 20% B for 2 min, linear gradient 20–80% B from 2 to 6 min and hold at 80% B for 3.5 min, then quickly returned to initial 20% B in 1.5 min and maintained for a further 2 min for column balance. Dehydrocholic acid was used as the internal standard (IS), and relative levels of Glu-CA and Glu-CDCA were expressed as peak area, normalized by dividing peak area of the IS. All experiments were conducted in triplicates. Assessment of mucosal damage and biochemical analysis Tissue sections (5 μm) were stained with haematoxylin and eosin. Histopathological scoring was performed by an experienced pathologist blinded to the experimental conditions, using an established semiquantitative score ranging from 0 to 6 based on infiltration of inflammatory cells and epithelial damage. Immunohistochemistry Tissue specimens were fixed in 10% formalin for 12–24 h, dehydrated and paraffin embedded. Standard immunohistochemical procedures were performed. Tissue sections were incubated with the primary antibody (rabbit polyclonal anti-FXR, 1:100; goat polyclonal anti-FGF15, 1:100; rabbit polyclonal anti-PPARα, 1:200) for 2 h at room temperature, followed by 30 min incubation with the pre-diluted horseradish peroxidase-conjugated secondary antibody (1:400). For negative controls, 1% non-immune serum in PBS replaced the primary antibodies. The immunohistochemistry staining of FXR, FGF15 and PPARα was scored by measuring the integrated optical density of at least three visions of each slice using Image pro-plus 6.0 software. Data are expressed as mean±s.e.m. of six mice. Quantitative reverse transcriptase PCR Total tissue and cell RNA extraction were performed using the RNAiso Plus reagent (TaKaRa Biotechnology Co., Ltd, Dalian, China) according to the manufacturer’s protocol. Complementary DNA was generated from 500 ng total RNA using SuperScript II Reverse Transcriptase (Invitrogen). Quantitative reverse transcriptase PCR analysis was carried out using SYBR green PCR mastermix and analysed on a MyIQ real-time PCR cycler (BioRad, Veenendaal, The Netherlands). Values were normalized to GAPDH. Sequences for primers and siRNA are listed in Supplementary Tables 2–5 . Western blot analysis Tissue extracts were prepared, subjected to SDS–PAGE using 8% gradient (Bis-Tris Midi Gel, Invitrogen) polyacrylamide gels and analysed by immunoblotting with antibody to CYP7A1 (1:500). Blots were stripped and reprobed with antibody to GAPDH (1:2,000) to normalize for protein load. Protein expression was quantified by densitometry using a Microtek ScanMaker i900 and FujiFilm Multiguage 3 software, and expression data were normalized to levels of the GAPDH loading control. UGT activity detection Tissues from six to eight mice were pooled and homogenized to make 20% homogenates in the 10 mM phosphate buffer containing 5 mM EDTA. The homogenates were subjected to centrifugation at 9,000 g for 20 min to isolate pooled post-mitochondrial fractions. The protein concentrations of the S9 were determined with BCA protein assay kit. All the S9 were stored at −80 °C before use [55] . The UGT activities were determined towards various substrates in pooled mice S9. A typical incubation mixture contained 50 mM Tris-HCl buffer (pH 7.4), 10 mM MgCl 2 , 25 μg ml −1 alamethicin, UDPGA, S9 and a selective substrate, including estradiol, CDCA, 4-MU, MPA or naloxone. S9 fractions were preincubated with alamethicin for 30 min at 4 °C. The concentrations of estradiol, CDCA, 4-MU, MPA and naloxone were 20, 50, 100, 200 and 20 μM, respectively, all of which were the concentrations below apparent Km values [20] , [56] . Other experimental conditions were the same as those described before [20] , [56] . The enzymatic activity was determined by HPLC and LC-MS analysis of the produced metabolites of the respective substrate [20] , [56] , [57] . Incubation conditions are listed in Supplementary Table 1 . Quantification of bile acids in mice The abundance of bile acids across multiple tissue compartments was assayed. Bile acids were extracted in 70% ethanol at 55 °C for 4 h, and bile salt species were analysed by the ultra-fast liquid chromatography (UFLC)-Triple-time of flight/MS analysis [58] , [59] . The alcoholic extracts were subjected to further solid-phase extraction using solid-phase extraction technique (UCT-CLEAN UP C18, Oasis-HLB and Oasis-MAX cartridges), and then the organic solvent was evaporated by Speed-Vac (Thermo Savant, Waltham, MA). The residue was reconstituted in 100 μl methanol by vortexing. The chromatographic system consisted of a Shimadzu (Kyoto, Japan) UFLC system performed on AB SCIEX Triple TOF 5,600 mass spectrometer equipped with an atmospheric pressure chemical ionization probe in a Turbo V ion source (AB Sciex). The chromatographic separation was carried out on a ZOEBAX Eclipse Plus C18 column (2.1 × 150 mm, 3.5 μm) (Agilent Technologies) and protected by a SecurityGuard (Phenomenex Inc., CA, USA). The mobile phase (delivered at 0.2 ml min −1 ) consisted of (A) 2.6 mmol l −1 ammonium acetate in water (adjusted to pH 6.8 with ammonium hydroxide) and (B) acetonitrile. The MS analysis was performed in a full negative scan mode from m / z 50 to 1,000 and the respective pseudomolecular ion [M–H] − for each bile acid species was extracted for quantification under extracted ion chromatogram mode. The information of fragment ions produced at Q3 was used to ascertain the identity of bile acid species. The retention time, pseudomolecuar ions and fragment ions for all the bile acids species are shown in Supplementary Table 6 . Analyst 1.4.2 software (AB Sciex) was used for system control, PeakView software for data exploration and quantification data were acquired with MultiQuant software 2.0. Quantification of OEA The extraction, purifcation and quantifcation of OEA were performed as described previously [60] . Intestinal contents were dounce-homogenized and extracted with chloroform/methanol/Tris–HCl 50 mmol l −1 pH 7.5 (2:1:1, vol/vol) containing IS (propranolol, 10 ng ml −1 ). The lipid-containing organic phase was dried down, weighed, and prepurifed by open-bed chromatography on silica gel. The prepurifed lipids were analyzed by liquid chromatography–atmospheric pressure chemical ionization–mass spectrometry by using a Shimadzu high-performance liquid chromatography apparatus (LC-10ADVP) coupled to a Shimadzu (LCMS-2010) quadrupole mass spectrometry via a Shimadzu atmospheric pressure chemical ionization interface. The chromatographic separation was achieved on an Agilent C18 column (150 × 2.1 mm, 3.5 μm) (Agilent Technologies, USA), protected by an SecurityGuard (Phenomenex Inc. CA. USA). The mobile phase comprising 0.1% formic-acid solution (A) and acetonitrile (B) was delivered at a flow rate of 0.25 ml min −1 using a gradient program set as: initial 30% B for 2 min, linear gradient 30–90% B from 3 to 5.5 min and to 95% B until 10 min, and then returned back to initial 30% in 2 min and maintained for a further 3 min for column balance. Selective ion monitoring was performed in the positive mode for the determination of pseudomolecular ions of OEA at m/z 326.2 and the IS propranolol at m / z 260.1. The amounts of OEA in tissues are expressed as micrograms per gram of wet tissue weight. Statistical analysis All experimental data are expressed as the mean±s.e.m. as indicated in the figure legends. Differences among multiple groups were tested using one-way analysis of variance followed by Dunnett’s post-hoc comparisons. Differences between two groups were tested by the Student’s t -test. Differences were considered significant if P <0.05 and have been marked with asterisks in the graph accordingly. How to cite this article: Zhou, X. et al . PPARα-UGT axis activation represses intestinal FXR-FGF15 feedback signalling and exacerbates experimental colitis. Nat. Commun. 5:4573 doi: 10.1038/ncomms5573 (2014).